Tumour-on-a-chip provides an optical window into nanoparticle tissue transport Nanomaterials are used for numerous biomedical applications, but the selection of optimal properties for maximum delivery remains challenging. Thus, there is a significant interest in elucidating the nano–bio interactions underlying tissue accumulation. To date, researchers have relied on cell culture or animal models to study nano–bio interactions. However, cell cultures lack the complexity of biological tissues and animal models are prohibitively slow and expensive. Here we report a tumour-on-a-chip system where incorporation of tumour-like spheroids into a microfluidic channel permits real-time analysis of nanoparticle (NP) accumulation at physiological flow conditions. We show that penetration of NPs into the tissue is limited by their diameter and that retention can be improved by receptor targeting. NP transport is predominantly diffusion-limited with convection improving accumulation mostly at the tissue perimeter. A murine tumour model confirms these findings and demonstrates that the tumour-on-a-chip can be useful for screening optimal NP designs prior to in vivo studies. There have been significant advancements in the chemical synthesis and design of cancer-targeting therapeutic and diagnostic agents. However, delivery of these agents remains inconsistent owing to poor control over the pharmacokinetics and accumulation of carrier systems in diseased tissues in vivo [1] . Overcoming this problem requires a better understanding of how blood-borne carriers enter their target tissue and distribute at the cellular level. In vivo animal models are useful for assessing general pharmacokinetics but make it impossible to evaluate tumour tissue transport independent of blood clearance rate, vascular permeability, tissue clearance and lymphatic drainage [2] . Animal studies are also hindered by the limited resolution of whole-animal imaging techniques which makes it difficult to visualize target tissues at the cellular level [3] . As a result, our knowledge of carrier–cellular interactions is predominantly gained from in vitro cell monolayer experiments [4] . These studies typically characterize the binding affinity, uptake, cellular responses and toxicity of these agents. [5] However, the lack of three-dimensional tissue architecture and dynamic flow conditions make these findings inaccurate in predicting in vivo outcomes. Microfluidic devices offer a highly customizable microscale platform to evaluate complex cellular configurations using microlitre amounts of reagents under controllable flow conditions [6] . Microfluidic devices can be used to culture cells [7] , create microenvironments [8] , mimic organs [9] or evaluate organ tissue ex vivo [10] . Several in vitro setups have been used to evaluate drug transport mechanisms but not for studying the role of drug carrier design in tumour transport. These previous studies do not provide a definitive conclusion on the effect of the physicochemical properties of a molecule or nanocarrier in mediating transport through a tumour tissue because most small organic drug molecules (for example, doxorubicin and paclitaxel) are within a narrow size range. Although there are various permutations of microfluidic chip designs for mimicking tumour systems and for analysing drug transport, none have been validated using animal models, and therefore, it is difficult to assess the accuracy of these microfluidic devices for predicting in vivo outcome. Nevertheless, such studies highlight microfluidics as potential strategy for the rapid and cost-effective pre-screening of drugs while also providing sufficient data to model the transport process prior to full animal studies [6] . The optimal microfluidic design to mimic in vivo tumour systems remains unclear but is a very active research area. It is well recognized that NP size, shape and surface chemistry can affect tumour accumulation [4] . However, the transport kinetics, NP retention and the role of interstitial flow rate within a tumour remain unclear. Here, our objective is to develop and apply a tumour-on-a-chip microfluidic platform to study the transport of synthetic carriers through a three-dimensional tissue environment. We use a tumour-on-a-chip system to evaluate the roles of NP diameter, receptor targeting and flow conditions on transport within a model tumour tissue. We demonstrate that NP tissue accumulation is restricted to hydrodynamic diameters of <110 nm with receptor targeting improving accumulation and retention. The flow rate of NPs only affected their accumulation at the tissue periphery and did not increase their penetration depth. These findings are confirmed in a murine xenograft model and demonstrate that the tumour-on-a-chip provides an accurate in vitro method to predict in vivo NP transport in MDA-MB435 tumour tissue. Tumour-on-a-chip characterization Our tumour-on-a-chip system consists of a multi-cellular spheroid immobilized in the channel of a two-layer polydimethylsiloxane (PDMS) microfluidic chip ( Fig. 1 ). The spheroid contains a heterogeneous distribution of MDA-MB-435 cells embedded in an extracellular matrix (ECM) forming a tortuous network of interstitial spaces similar to the tumour tissue. Spheroids are frequently used to screen the therapeutic efficiency of drugs, antibodies and NPs in a static environment [2] , [11] , [12] . Incorporation of the spheroid into a microfluidic chip holds the micro-tissue stationary in moving solution, generates controllable flow conditions and provides an optical window for non-disruptive real-time analysis using confocal microscope imaging [13] . First, we prepared 280 μm MDA-MB-435 melanoma cell spheroids and gently loaded them into the PDMS chip using gravity-driven flow. Cells inside the spheroid remained viable, and measured 10.69±2.67 μm in diameter at the rim and 12.61±2.63 μm in deeper layers ( Supplementary Fig. S1 ). Interstitial spaces between the cells measured 1.00±0.52 μm and represented 16.23±2.47% of the total spheroid volume. A non-uniform layer of ECM containing laminin protein surrounds the spheroids and forms a physical barrier between the cells and their surrounding medium. Regulating the volumetric flow rate into the microfluidic device creates the unique flow properties necessary for precise control of the pressure gradient, shear stress and fluid velocity in the channel ( Supplementary Fig. S2 ). Flow rates between 50 and 450 μl h −1 produced a 75–675 μm s −1 fluid velocity ( Fig. 1c ), which is comparable to blood flow in tissue capillaries [14] , [15] . At 450 μl h −1 , flow remained laminar with the pressure drop at 9 Pa and shear stress at 0.06 Pa in the imaging chamber where the spheroid is immobilized. When flow rate is raised from 50 to 450 μl h −1 , accumulation kinetics of 10 kDa dextran demonstrate that convective flow increases from 0.4 to 1.41 μm s −1 . These values are similar to interstitial flow inside a tumour, which can vary between 0.1 and 3 μm s −1 (refs 16 , 17 ). The tumour-on-a-chip therefore provides an experimental platform with controllable interstitial flow through a three-dimensional tissue. 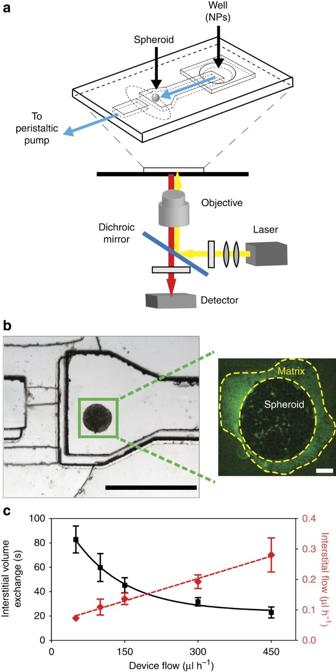Figure 1: Schematic and characterization of the tumour-on-a-chip. (a) Schematic of the PDMS microfluidic device on a microscope stage. (b) Image of the microfluidic device (left) demonstrating that channel width is 600 μm at the inlet then widens to 1,200 μm in the imaging chamber where the spheroid is immobilized. Channel height is 250 μm and then drops to 25 μm at the end of the imaging chamber forming a dam; scale bar, 1,000 μm. A spheroid (right) stained with anti-Laminin-FITC for 10 min and then flushed with imaging media for 5 min; scale bar, 100 μm. (c) Flow rate versus media exchange (black squares) which represents the amount of time required for the non-fluorescent media inside the spheroid to be filled with 10 kDa Dextran-568. The corresponding interstitial flow rates (red diamonds) are displayed. Error bars represent s.e.m. wheren=3 spheroids. Figure 1: Schematic and characterization of the tumour-on-a-chip. ( a ) Schematic of the PDMS microfluidic device on a microscope stage. ( b ) Image of the microfluidic device (left) demonstrating that channel width is 600 μm at the inlet then widens to 1,200 μm in the imaging chamber where the spheroid is immobilized. Channel height is 250 μm and then drops to 25 μm at the end of the imaging chamber forming a dam; scale bar, 1,000 μm. A spheroid (right) stained with anti-Laminin-FITC for 10 min and then flushed with imaging media for 5 min; scale bar, 100 μm. ( c ) Flow rate versus media exchange (black squares) which represents the amount of time required for the non-fluorescent media inside the spheroid to be filled with 10 kDa Dextran-568. The corresponding interstitial flow rates (red diamonds) are displayed. Error bars represent s.e.m. where n =3 spheroids. Full size image Effect of NP size on tissue accumulation With the tumour-on-a-chip we addressed a series of questions concerning NP tumour delivery that have been difficult to address using conventional animal models or cell culture experiments. In the first set of experiments, we examined the effect of NP size on tissue transport kinetics. Fluorescently labelled PEGylated gold NPs [18] possessing a hydrodynamic diameter of 40, 70, 110 or 150 nm ( Supplementary Table S1 and Supplementary Fig. S3 ) were administered to spheroids in the microfluidic chip for 1 h at 50 μl h −1 ( Fig. 2 ) and accumulation was quantified ( Supplementary Fig. S4 ). Of note, we have previously characterized the distance-dependent quenching effect of fluorescent molecules on the surface of gold NPs and used these results as guidelines for the design of the current NPs to ensure adequate fluorescence for our studies [17] . The 40 and 70 nm NPs were visible inside the spheroid’s interstitial spaces within 10 min and showed an entry rate of 0.00400, min −1 and 0.00396, min −1 , respectively ( Supplementary Fig. S5 ). In contrast, the 110 and 150 nm NPs were excluded from interstitial spaces and accumulated significantly less. Efflux of the NPs from the spheroid tissue occurred rapidly and confirms that NP PEGylation inhibits binding to cells and ECM proteins ( Supplementary Fig. S6 ). Electron microscopy and spheroid silver staining were used to confirm the presence of PEG-NPs ( Supplementary Fig. S7 ). However, the multiple washes required for sample preparation removed PEG-NPs from the spheroid and made it impossible to quantify accumulation. 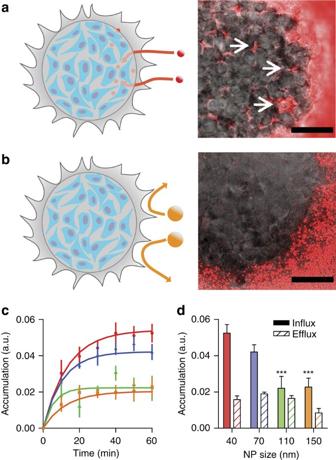Figure 2: Effect of NP size on tissue accumulation. (a) Schematic (left) and image (right) of 40 nm fluorescent PEG-NPs administered for 1 h at 50 μl h−1entering the spheroid and accumulating in the interstitial spaces (arrows). Scale bar, 100 μm. (b) Schematic (left) and image (right) of 110 nm fluorescent PEG-NPs administered for 1 h at 50 μl h−1being excluded from the spheroid. Scale bar, 100 μm. Images inaandbrepresent an overlay of fluorescence (excitation: 633 nm, emission: 650–700 nm) and differential interference contrast images. (c) Tissue accumulation of different 40 (red), 70 (blue), 110 (green) and 150 nm (orange) PEG-NPs administered to the spheroid at 50 μl h−1. (d) Tissue accumulation of PEG-NPs after 1 h at 50 μl h−1and after flushing with clear solution for 30 min at 50 μl h−1. Tissue accumulation represents the average fluorescent intensity from the spheroid’s perimeter to a depth of 75 μm normalized to the medium’s fluorescence. Data is presented as the average values from three to five spheroids with s.e.m. ***P<0.001 using ANOVA. Figure 2: Effect of NP size on tissue accumulation. ( a ) Schematic (left) and image (right) of 40 nm fluorescent PEG-NPs administered for 1 h at 50 μl h −1 entering the spheroid and accumulating in the interstitial spaces (arrows). Scale bar, 100 μm. ( b ) Schematic (left) and image (right) of 110 nm fluorescent PEG-NPs administered for 1 h at 50 μl h −1 being excluded from the spheroid. Scale bar, 100 μm. Images in a and b represent an overlay of fluorescence (excitation: 633 nm, emission: 650–700 nm) and differential interference contrast images. ( c ) Tissue accumulation of different 40 (red), 70 (blue), 110 (green) and 150 nm (orange) PEG-NPs administered to the spheroid at 50 μl h −1 . ( d ) Tissue accumulation of PEG-NPs after 1 h at 50 μl h −1 and after flushing with clear solution for 30 min at 50 μl h −1 . Tissue accumulation represents the average fluorescent intensity from the spheroid’s perimeter to a depth of 75 μm normalized to the medium’s fluorescence. Data is presented as the average values from three to five spheroids with s.e.m. *** P <0.001 using ANOVA. Full size image Effect of receptor targeting on tissue accumulation Next, we used the tumour-on-a-chip to compare passive- and active-targeting NPs. Passive NPs are predominantly conjugated with PEG to minimize interactions with cell receptors and other proteins. They are designed to evade blood clearance and progressively diffuse into tumours [19] . The 40 nm PEG-NPs were used as models of passive-targeting NPs and they diffused into the surrounding ECM reaching 27.37±6.02% of the administered dose after 1 h. Average fluorescence in the spheroid was significantly lower at 4.98±0.23% and mostly limited to interstitial spaces ( Fig. 3a,b ). With active-targeting NPs, the addition of a receptor-targeting biomolecule can increase accumulation compared with diffusion alone. NPs functionalized with the iron-transporting transferrin (Tf) protein were used as a model of active-targeting NPs and formed a concentrated region at the spheroid perimeter 287.1±101.2% of the administered dose ( Fig. 3c,d ). This highly fluorescent ‘binding-site barrier’ is caused by an elevated accumulation of NPs in the outermost ECM and Tf receptor-expressing cells ( Supplementary Fig. S8 ). Inside the spheroid, Tf-NPs co-localized with the cells and formed visible punctate regions caused by receptor binding [20] ( Fig. 3c ). Tf-NPs showed a 15-fold increase inside the spheroids compared with PEG-NPs similar to certain tumour regions in vivo [3] . Flushing produced a slight decrease in peripheral ECM fluorescence but not in spheroid fluorescence. Blocking the cell receptors with soluble Tf protein reduced the accumulation inside the spheroid by 50% but did not affect the surrounding ECM ( Supplementary Fig. S9 ). This suggests that a combination of specific interactions with cell receptors and non-specific protein interactions with ECM proteins anchor the Tf-NPs in the tissue preventing efflux. Electron microscopy and spheroid silver staining confirmed the presence of a binding-site barrier with Tf-NPs bound to cell membranes and the surrounding ECM ( Supplementary Figs S10, S11 ). However, we detected minimal Tf-NPs inside the cells. These findings illustrate that the addition of Tf to the 40 nm NP surface improves accumulation and retention in the tissue through receptor-specific and non-specific protein interactions. 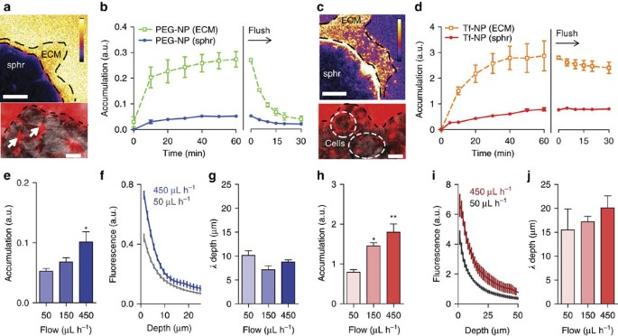Figure 3: Effect of NP functionalization and flow rate. (a) Intensity map (top) of PEG-NP fluorescence taken at 40X after 1 h of flow at 50 μl h−1. Image (bottom) of PEG-NP fluorescence in the interstitial spaces (arrows). Scale bars, 50 μm. (b) Mean fluorescence of surrounding matrix (ECM) and spheroid (sphr) treated with PEG-NPs at 50 μl h−1. (c) Intensity map (top) of Tf-NP fluorescence taken after 1 h of flow at 50 μl h−1. Image (bottom) of Tf-NP punctuate fluorescence co-localizing with cell membranes. Scale bars, 50 μm. (d) Mean fluorescence of surrounding matrix and spheroid treated with Tf-NPs at 50 μl h−1. Mean spheroid fluorescence (e), fluorescence distribution (f) and penetration depth (g) of spheroids treated with PEG-NPs at various flow rates. Mean spheroid fluorescence (h), fluorescence distribution (i) and penetration depth (j) of spheroids treated with Tf-NPs at various flow rates. Data are presented as the average values from three to five spheroids with s.e.m. *P<0.05, **P<0.01 using ANOVA. Figure 3: Effect of NP functionalization and flow rate. ( a ) Intensity map (top) of PEG-NP fluorescence taken at 40X after 1 h of flow at 50 μl h −1 . Image (bottom) of PEG-NP fluorescence in the interstitial spaces (arrows). Scale bars, 50 μm. ( b ) Mean fluorescence of surrounding matrix (ECM) and spheroid (sphr) treated with PEG-NPs at 50 μl h −1 . ( c ) Intensity map (top) of Tf-NP fluorescence taken after 1 h of flow at 50 μl h −1 . Image (bottom) of Tf-NP punctuate fluorescence co-localizing with cell membranes. Scale bars, 50 μm. ( d ) Mean fluorescence of surrounding matrix and spheroid treated with Tf-NPs at 50 μl h −1 . Mean spheroid fluorescence ( e ), fluorescence distribution ( f ) and penetration depth ( g ) of spheroids treated with PEG-NPs at various flow rates. Mean spheroid fluorescence ( h ), fluorescence distribution ( i ) and penetration depth ( j ) of spheroids treated with Tf-NPs at various flow rates. Data are presented as the average values from three to five spheroids with s.e.m. * P <0.05, ** P <0.01 using ANOVA. Full size image Effect of flow rate on tissue accumulation Finally, we wanted to investigate how interstitial flow rates affected NP accumulation. Variable convection is a common feature of the tumour environment and can be attributed to heterogeneous vascularization, interstitial pressure and lymphatic drainage. These conditions produce rapid interstitial flow at the tumour perimeter and no convection in the centre [17] . Augmenting the flow rate in our microfluidic device from 50 to 450 μl h −1 produced a two-fold increase in both PEG-NPs and Tf-NPs accumulation ( Fig. 3e–j ). We originally hypothesized that faster flow rates would increase convection, which allowed NPs to penetrate deeper in the tissue. However, it was the amplitude of tissue fluorescence that increased with no detectable change in the average penetration depth ( Fig. 3g,j ). Instead, faster flow rates produced a higher accumulation of NPs on the spheroid’s outer layer and increased the total number of NPs diffusing into the tissue ( Supplementary Fig. S12 ). These findings demonstrate that interstitial flow determines the number of NPs accumulated at the tissue interface. Once at the interface, the NPs are immobilized by the ECM fibres and diffuse into the tissue over time. In vivo tumour accumulation We used a murine xenograft MDA-MB-435 tumour model [18] , [19] to evaluate whether the tumour-on-a-chip system predicted the tissue transport of NPs through the same tumour cells in vivo ( Fig. 4 ). We intravenously injected two different sized fluorescently labelled PEG-NPs (50 versus 160 nm) and a fluorescently labelled 50 nm Tf-NPs into tumour-bearing mice. Whole animal imaging reveals minimal tumour accumulation for 160 nm PEG-NP, whereas 50 nm PEG-NPs and 50 nm Tf-NPs progressively accumulate between 2 and 48 h ( Fig. 4a,b ). At 48 h post-injection, we isolated the tumour tissue, silver stained the tissues to highlight NP location and measured the penetration depth of the different NP designs. Histological analysis demonstrates that 160 nm PEG-NPs are seldom found in the tumour tissue and do not penetrate into the tissue surrounding tumour vasculature. This is in agreement with our tumour-on-a-chip data where NPs larger than 100 nm did not penetrate into the spheroid tissue after 1 h ( Fig. 2b ). For 50 nm NPs, the addition of Tf increased accumulation of NPs in the tissue surrounding the blood vessel ( Fig. 4c ). Statistical analysis demonstrates a significant increase in the accumulation of 50 nm Tf-NPs within a 7 μm radius of tumour blood vessels. These findings confirm the tumour-on-a-chip results which demonstrates that NP design is an important determinant of tissue transport. The accumulation is limited to NPs with diameters that are <110 nm and significantly increased by active targeting in MDA-MB-435 tumours for the 40 nm NPs. 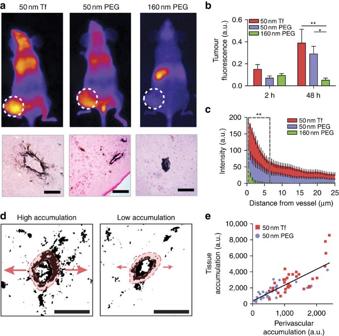Figure 4:In vivobehaviour of NPs. (a) Representative images (top) of tumour fluorescence from mice injected with NPs in the tail vein at 48 h post-injection and sample images (bottom) of tumour histological sections treated with a silver enhancement kit to visualize NPs around blood vessels. The 50 nm Tf-NPs and 50 nm PEG-NPs diffuse into the tissue, whereas 160 nm PEG-NPs remain inside the blood vessel. Scale bars, 50 μm. (b) Quantification of animal fluorescence at 2 and 48 h using whole animal images (Data are presented as the average fluorescence and s.e.m wheren=3 mice; *P<0.05, **P<0.01 using two-way ANOVA). (c) Distribution of NPs in tumour blood vessels quantified using image analysis of silver-stained histological sections (Data are presented as the average silver stain intensity and s.e.m wheren=32 for 50 nm Tf-NP,n=31 for 50 nm PEG-NPs, andn=15 for 160 nm PEG-NPs where n is the number of blood vessels analyzed; **P<0.01 using two-way ANOVA). (d) Representative image of two distinct blood vessels in the same tumour treated with 50 nm PEG-NP demonstrating variability in extravasation and tissue penetration. Image threshold was set to isolate silver-stained NPs in the tissue. Red highlighted area corresponds to the perivascular region. Scale bars, 25 μm. (e) Correlation between accumulation of NPs in the perivascular region (5 μm radius) and the tumour tissue (25 μm radius) around the blood vessel. Figure 4: In vivo behaviour of NPs. ( a ) Representative images (top) of tumour fluorescence from mice injected with NPs in the tail vein at 48 h post-injection and sample images (bottom) of tumour histological sections treated with a silver enhancement kit to visualize NPs around blood vessels. The 50 nm Tf-NPs and 50 nm PEG-NPs diffuse into the tissue, whereas 160 nm PEG-NPs remain inside the blood vessel. Scale bars, 50 μm. ( b ) Quantification of animal fluorescence at 2 and 48 h using whole animal images (Data are presented as the average fluorescence and s.e.m where n =3 mice; * P <0.05, ** P <0.01 using two-way ANOVA). ( c ) Distribution of NPs in tumour blood vessels quantified using image analysis of silver-stained histological sections (Data are presented as the average silver stain intensity and s.e.m where n =32 for 50 nm Tf-NP, n =31 for 50 nm PEG-NPs, and n =15 for 160 nm PEG-NPs where n is the number of blood vessels analyzed; ** P <0.01 using two-way ANOVA). ( d ) Representative image of two distinct blood vessels in the same tumour treated with 50 nm PEG-NP demonstrating variability in extravasation and tissue penetration. Image threshold was set to isolate silver-stained NPs in the tissue. Red highlighted area corresponds to the perivascular region. Scale bars, 25 μm. ( e ) Correlation between accumulation of NPs in the perivascular region (5 μm radius) and the tumour tissue (25 μm radius) around the blood vessel. Full size image In our microfluidic studies, we demonstrated that properties of the tumour microenviroment such as interstitial flow rates can also affect NP transport into the tissue. Our in vitro findings revealed that the number of NPs at the spheroid–media interface reflected total tissue accumulation ( Fig. 3e–j and Supplementary Fig. S12 ). To validate if a similar relationship was apparent in vivo , we took advantage of the large variability in tissue accumulation of NPs between different blood vessels. For a given tumour, NPs can accumulate around blood vessels at different quantities ( Fig. 4d ). Using histological data from tumours treated with 50 nm Tf-NPs and 50 nm PEG-NPs, we compared the accumulation of NPs at the blood vessel–tumour tissue interface with accumulation in deeper cell layers surrounding the blood vessel. We defined the blood-vessel interface or ‘perivascular region’ as the region within a 5 μm radius of the blood vessel and determined its relationship with the accumulation within a 25 μm radius. Figure 4e demonstrates a linear trend between the perivascular region and tumour tissue accumulation. We used the F test to confirm that the positive slope was significantly different from the null hypothesis ( P <0.0001). This finding is in agreement with our tumour-on-a-chip results demonstrating that higher flow rates increased the concentration of NPs at the spheroid surface. However, because we cannot directly characterize the flow, permeability, pressure differential, porosity and other properties of the tumour microenvironment in vivo , our in vivo conclusions remain correlative in nature. Our tumour-on-a-chip system allowed us to investigate the transport mechanism of NPs through a model tissue. The peripheral matrix surrounding the spheroid is analogous to the laminin-rich basement membrane through which plasma must diffuse prior to entry into the tissue. Similarly, liquid in the tumour-on-a-chip travels at physiological rates, encounters the peripheral matrix and produces convection through the spheroid’s interstitial spaces. Our data demonstrate that both NP physicochemical properties and the tumour microenvironment can affect tissue accumulation. Our study illustrates that tissue transport requires the NPs to embed into the tissue–fluid interface and progressively diffuse into the tissue. For passive targeting, the reservoir at the tissue–fluid interface is responsible for dictating the number of NPs diffusing into the tissue. For active targeting, the binding-site barrier will saturate available binding sites and allow additional NPs to diffuse into the tissue. Our findings in vitro and in vivo reveal that the concentration of NPs in the reservoir or the binding-site barrier is an important determinant of tissue transport kinetics. These conclusions are in agreement with models of inconsistent NP delivery due to the variable tumour vasculature [21] . The tissue–fluid interface appears to predict NP tumour accumulation in vivo . Interestingly, previously studies show a time-dependent increase in NPs at the spheroid surface, correlated with overall tissue accumulation [12] , [22] . The tumour-on-a-chip reveals that interstitial flow rate, cell receptor binding and NP diameter all influence accumulation at the tissue–media interface. At the interface, NPs <110 nm can diffuse through the ECM and interact with tumour cells. Above 110 nm, NPs are excluded from the MDA-MB-435 spheroids and the tumours because they are larger than the ECM’s effective pore size and cannot embed into the protein matrix. Our findings are in agreement with previous studies demonstrating the limited tissue penetration of larger NPs [19] , [21] , [23] , [24] . A recurring 100 nm cutoff may reflect the upper limit of ECM diffusivity. The addition of Tf to the NP surface produced a 15-fold increase in the accumulation of Tf-NPs relative to PEG-NPs. Unfortunately, receptor targeting does not benefit from such an impressive advantage in vivo . Systemically administered Tf-NPs show better tumour transport kinetics around blood vessels, but this did not translate into a statistically significant increase in tumour fluorescence. This may be due to several factors including large inter-animal variability, the addition of PEG to the 50 nm Tf-NPs to prevent blood clearance and numerous NP-biological interactions upstream of tumour accumulation. Our tumor-on-a-chip data also suggest that the challenges of receptor targeting include non-specific binding to the ECM and formation of a binding-site barrier. Previous work has demonstrated that the receptor targeting can produce a moderate increase in tumour accumulation [25] but may only benefit NPs <40 nm when entering specific ‘slow flow’ regions of the tumour [3] . When NPs are directly administered into the tumour, receptor targeting can improve therapeutic outcome [26] . Whether active targeting is only useful in certain regions of the tumour or whether it impedes upstream events such as blood clearance and extravasation remains an important question in drug delivery. In regards to tissue transport, short-term experiments with systems like the tumour-on-a-chip can predict the long-term tissue transport of NPs when coupled to highly sensitive detection techniques such as confocal microscopy. With rapid 1 h in vitro experiments, we successfully predicted NP transport in MDA-MB-435 in vivo tumours. It must still be confirmed whether this approach can predict drug carrier behaviour in vivo using other tumour cell lines and other tissue models. The tumour-on-a-chip improves on previous in vitro work where spheroids remained in a static solution for several hours [2] , [11] , [12] , [24] and required disruption before [8] or after [2] , [11] , [12] , [24] incubation with drug carrier systems. The real-time imaging of intact spheroids using confocal microscopy improved sensitivity and provided a window into early NP–tissue interactions. These improvements offer an unprecedented look at early NP–tissue interactions under controllable flow conditions. Our experimental set-up permits the rapid assessment of how a NP’s physicochemical properties affect its transport through tumours and potentially, other tissues. On the basis of this initial study, early NP–tissue interactions monitored using microfluidic-based tissue models may successfully predict the long-term behaviour of NPs in a tissue in vivo . With recent advances in the commercialization of microfluidics and nanomaterials, researchers can simply insert their specific tumour model into a purchased device. This will facilitate the evaluation of multiple NP designs in different tumour systems and will validate microfluidic-based tissue models as versatile platforms to evaluate the performance of drug carriers prior to animal studies. Future iterations of our device can include additional compartments to mimic blood filtration by the liver and kidneys to better predict the systemic behaviour of NPs. Alternatively, future designs could produce a high-throughput system by running channels in parallel to screen large libraries of NP designs for optimal tumour targeting. A high-throughput system provides a means for accelerating the development of therapeutic nanomaterials by selecting the most promising candidates to evaluate in vivo . Finally, a tumour-on-a-chip design which permits the analysis of patient tumour biopsies could also be used to predict the therapeutic outcome of NP-treatment. Fluorescent NP synthesis The 15 nm gold NPs were synthesized by citrate reduction method. The 30, 70 and 100 nm AuNPs were synthesized using hydroquinone-mediated growth of the 15 nm seeds [27] . Size and polydispersity was verified for each batch using a Zetasizer Nano ZS 633 nm instrument (Malvern). AuNPs were washed three times using 340 μM sodium citrate tri-basic (Ci) and functionalized with PEG (Laysan) or Tf (Sigma). PEG-NPs were prepared by adsorbing a mixture of 15% NH 2 -PEG-5k-SH and 85% CH 3 -PEG-5k-SH to 15 nm NPs for 1 h at 60 °C (ref. 18 ). For 30, 70 and 100 nm, we used the same conditions with 15% NH 2 -PEG-10k-SH and 85% CH 3 -PEG-10k-SH. The longer PEG was necessary to prevent gold NP-mediated quenching of fluorescence [18] . PEG-NPs were centrifuged and washed twice with 0.02% Tween-20+340 μM Ci buffer (Sigma), washed once with 340 μM Ci buffer and incubated with Cyto633-NHS ester (Cytodiagnostics) overnight at 4 °C. PEG-NPs were centrifuged and washed three times as described in the previous step. The initial intent was to normalize NP dose to administer the same surface area as 25 nM of 15 nm NPs for the larger sizes. However, owing to higher scattering and overall optical density of the NP solutions it was difficult to detect signal fluorescence. When we diluted the ~1/200 NPs, we were able to achieve high fluorescence and used these dilutions indicated in Supplementary Table S1 . Cyto633-Tf was prepared by incubating Cyto633-NHS ester at a 10-to-1 molar excess with Tf in 200 mM carbonate buffer pH 8.3. The reaction was incubated at 4 °C overnight and purified twice using a NAP-5 desalting column (GE Healthcare) equilibrated in 0.1X PBS. The dye-to-protein ratio was ~5 as determined by ultraviolet–visible spectrometry according to the manufacturer’s instructions. Tf-Cyto-633 conjugate was still functional as it could bind to Tf-receptor expressing cells as assessed by flow cytometry. Binding of the Tf-Cyto-633 conjugate was blocked by native Tf protein at a 1:1 molar ratio. The Tf-NPs were functionalized by passive adsorption with Cyto633-labelled Tf for 1 h at 37 °C and washed three times in 340 μM Ci buffer+0.1% serum albumin. We checked for the stability of Tf-NPs by incubating the NPs in imaging media for 1 h and did not detect and desorption of Tf from the NP surface ( Supplementary Fig. S13 ). Cell culture conditions Spheroids were prepared with MDA-MB-435 cells (ATCC) as previously described [28] . Briefly, round-bottom 96-well plates were coated with polyhydroxyethyl methacrylate (Sigma), 750–1,500 cells were placed in each well and centrifuged at 800 g for 10 min. Spheroids were grown for 3 days in RPMI supplemented with 10% fetal bovine serum and 2.5% basement membrane extract (BD Matrigel) and measured using optical microscopy. Spheroids measuring 260–280 μm were loaded into microfluidic devices and used for experiments. Microfluidic device fabrication Microfluidic devices were fabricated with PDMS (Dow-Corning) as previously described [13] . The cured mould was removed from the epoxy resin master and irreversibly bonded to a 24 × 50 mm cover slip (VWR Scientific) using oxygen plasma (Harrick Scientific). Tygon tubing was inserted directly into the cored-out port holes. Microfluidic device was designed with a channel height of 250 μm to slightly compress the ~280 μm spheroids against the glass cover-slip to ensure adequate immobilization and optical definition. The channel entrance is 600 μm wide and widens further to 1,200 μm at the imaging chamber to reduce the fluid linear velocity and ensure gentle motion of spheroids before arriving at the dam wall to minimize physical damage. The width of the imaging chamber also allows solution to flow around the spheroid to induce a pressure drop across the tissue and generate convective flow through the tissue [13] . Spheroids were gently loaded into the microfluidic device using gravitational flow of imaging media (0.2% bovine albumin, 125 mM NaCl, 5.7 mM KCl, 2.5 mM CaCl 2 , 1.2 mM MgCl 2 , 10 mM HEPES and pH 7.4) [29] . Interstitial flow rates ( Supplementary Fig. S14 ) were quantified by measuring the time required to fill the interstitial space with 0.1 mM 10 kDA Dextran-568 (Invitrogen). An image was taken every second while dextran was flowed into the device. We measured the time between the appearance and disappearance of the non-fluorescent ‘tail’ exiting the spheroid [13] ( Supplementary Fig. S14 ). Administration of dextran at the various flow rates was performed on three separate spheroids. For ECM staining we used 10 μg ml −1 anti-Laminin-FITC (Abcam). Confocal microscope conditions The microfluidic device was mounted on a microscope stage inside a 37 °C incubator (Okolabs). Flow rate was controlled using a syringe pump. NP accumulation images were taken using a 40X or 63X oil emersion objectives at a 633 nm excitation and 650–700 nm emission on a Zeiss LSM710 confocal microscope. Images were taken at 10 μm depth intervals every 5–10 min for 1 h. Fluorescence distribution was analysed in ImageJ by drawing a contour around the spheroid freehand and a macro was developed to measure the mean fluorescence at various depths throughout the spheroid (1.38 μm increments of radial contraction). Accumulation was obtained by taking the mean fluorescence in the first 75 μm and normalizing to fluorescence of the surrounding media ( Supplementary Fig. S4 ). For each spheroid four separate Z-plane images were averaged per time point. All experiments were performed on at least three spheroids. Silver staining procedure For each experimental condition, 20–30 spheroids were harvested from 96-well plate into 1.5 ml tubes and treated with 25 nM PEG-NP or Tf-NP. Spheroids were washed once with PBS, fixed with 10% buffered formalin solution and embedded in low melt 3% agarose solution. Spheroids were then embedded in paraffin, sectioned, stained with hematoxylin, eosin and silver staining kit (Ted Pella). Samples were analysed by optical microscope and NP accumulation was determined by obtaining the sum intensity of silver stain in each spheroid section. Statistical analysis parameters All values in the Results and Discussion sections are presented as ‘mean value±s.d.’ The data in figures is presented as the average of at least three spheroids with s.e.m. Statistical significance was determined using ANOVA followed by the Dunnet post-test comparing all sizes to 40 nm or all flow rates to 50 μl h −1 . In vivo tumour model specifications To inoculate tumours, MDA-MB-435 cells collected by cell scraping, concentrated by centrifugation, resuspended in 50% Matrigel (BD) and 3 × 10 6 cells in 150 μl were injected subcutaneously into the mammary fat pad on the flank of 6-week-old female CD1 nude athymic mice (Charles River) and allowed to grow for three weeks. Mice bearing tumours with a 1 cm cross-sectional diameter were tail-vein injected with each NP formulation ( Supplementary Table S2 ). The quantity of NPs injected was normalized to achieve a surface area of 7 × 10 15 nm 2 . Tumour fluorescence was then monitored by whole animal fluorescence using a Carestream In Vivo FX Imager under isofluorane-enriched oxygen. Dorsal images of mice were taken at 0.17, 2 and 48 h post-injection at a 10 min exposure with excitation and emission wavelengths of 750 and 830 nm, respectively. Tumour accumulation of NPs was assessed using a method published by Chou and Chan [18] . Briefly, mean fluorescence of the tumour and opposing mouse flank were measured and normalized to their initial fluorescence at 0.17 h post-injection. Normalized flank fluorescence was then subtracted from normalized tumour fluorescence. Tumours were harvested from mice 48 h post-injection, fixed with formalin, sectioned at a thickness of 4 μm and stained with haemotoxylin-eosin as well as silver enhancement kit to visualize tissue features and NPs [30] , respectively. Stained sections were analysed by bright-field at 20X magnification on an Olympus IX-51 with an Amscope MU500 camera. NP distribution expanding radially away from blood vessels was analysed in ImageJ by drawing a contour around blood vessels freehand and a macro was developed to measure mean NP content at various radii into the tissue (0.5 μm increments of radial expansion). Interstitial flow rates Image analysis reveals that ~15% of a spheroid’s volume is its interstitial space. For a spheroids 280 μm in diameter, the volume of the interstitial space is 1.72 × 10 −12 m 3 . Because the interstitial spaces are heterogeneous in shape and dimensions, it is impossible to obtain the area of each space’s cross section. Instead, we modelled the interstitial space as a network of 1 μm channels that pass through the centre of the spheroid. The length of each ‘interstitial channel’ in this model is equal to the spheroid diameter (280 μm). This organization will produce 100% flow through channels in parallel with the microfluidic flow and 0% flow in perpendicular channels ( Supplementary Fig. S15 ). This concentric symmetry will produce an average flow efficiency of 50%. In a sphere, we need to consider all three planes, so the overall flow efficiency is 50% in each plane totalling 12.5%. Assuming that the shape and orientation of the interstitial channels remain constant regardless of the pump’s flow rates, the cross-sectional area ( A ) of each channel is shown in equation (1), and the volume ( V ) of each channel is shown in equation (2): In our spheroids, interstitial space represents 1.72 × 10 −12 m 3 and this translates into 7,836 channels with 12.5% flow efficiency ( E ). The average flow rate ( Q ) through each channel is shown in equation (3). where Q S is the flow through the spheroid which was determined experimentally using 10 kDa Dextran-568. Once the flow rate through the interstitial channels is obtained, it is possible to convert it to a velocity ( v ) using equation (4), which was used to produce Supplementary Table S3 and Fig. 1c . Calculating the rate of NP accumulation Flow of NPs in the microfluidic channel where a spheroid is held stationary causes a diffusion of NPs into the tissue. Once in the spheroid, the NPs can accumulate in or leave the tissue. In this context, the spheroid can be viewed as one functional unit with inputs and outputs, as shown in Supplementary Fig. S16 . On the basis of Supplementary Fig. S16 , a mathematical model can now be developed that accounts for the incoming and outgoing activities in the spheroid. It can be assumed that the rates at which NPs enter and leave the spheroid are proportional to the concentrations of NPs present in inlet reservoir and spheroid, respectively. Therefore, the time dependent value of NP accumulation in the spheroid is the resultant of the inputs and outputs. Putting these notions together yields equation (5). The concentration of NPs in the inlet reservoir ( C D ) remains constant independent of time; one can therefore simplify the equation for C S by normalizing it to C D (dividing both sides of equation (5) by C D ), as shown by equation (6): where C S is the concentration of NPs, which is normalized to C D , accumulated in the spheroid (dimensionless), k IN is the rate constant at which the NPs enter the spheroid (min −1 ), k OUT is the rate constant at which the NPs leave the spheroid (min −1 ), t is the independent variable, time (min). Equation (6) is a linear first-order differential equation with one dependent variable with respect to time, C S . Solving equation (6) via the integrating factor, exp (∫ k OUT d t ) or exp( k OUT t ) yields equation (7): Equation (7) has two rate constants. To solve for them empirically, one can substitute two experimental data points for ( C S , t ) into equation (7) and solve for the resulting set of two linear equations with two variables, k IN and k OUT . How to cite this article: Albanese, A. Tumour-on-a-chip provides an optical window into nanoparticle tissue transport. Nat. Commun. 4:2718 doi: 10.1038/ncomms3718 (2013).